Differentiation of multipotent vascular stem cells contributes to vascular diseases It is generally accepted that the de-differentiation of smooth muscle cells, from the contractile to the proliferative/synthetic phenotype, has an important role during vascular remodelling and diseases. Here we provide evidence that challenges this theory. We identify a new type of stem cell in the blood vessel wall, named multipotent vascular stem cells. Multipotent vascular stem cells express markers, including Sox17, Sox10 and S100β, are cloneable, have telomerase activity, and can differentiate into neural cells and mesenchymal stem cell-like cells that subsequently differentiate into smooth muscle cells. On the other hand, we perform lineage tracing with smooth muscle myosin heavy chain as a marker and find that multipotent vascular stem cells and proliferative or synthetic smooth muscle cells do not arise from the de-differentiation of mature smooth muscle cells. In response to vascular injuries, multipotent vascular stem cells, instead of smooth muscle cells, become proliferative, and differentiate into smooth muscle cells and chondrogenic cells, thus contributing to vascular remodelling and neointimal hyperplasia. These findings support a new hypothesis that the differentiation of multipotent vascular stem cells, rather than the de-differentiation of smooth muscle cells, contributes to vascular remodelling and diseases. Vascular diseases are a leading cause of death in many countries. The development of vascular diseases, such as intimal hyperplasia and atherosclerosis, involves proliferation and migration of vascular cells [1] , [2] , [3] , [4] . Vascular smooth muscle cells (SMCs) are the predominant cell type in the tunica media of the blood vessel wall. Studies from many laboratories have shown that cultured SMCs and SMCs in the neointima 'lose' the expression of smooth muscle myosin heavy chain (SM-MHC), a marker of contractile SMCs, and become proliferative and synthetic [5] , [6] , [7] , [8] , [9] , [10] . A widely accepted explanation is that SMCs have phenotypic plasticity and that mature or contractile SMCs can de-differentiate into proliferative and synthetic SMCs [4] , [11] , [12] , [13] . However, this de-differentiation process has not been directly demonstrated by tracking the fate of mature or contractile SMCs. Over the past decade, several types of SMC-related vascular progenitors in the blood vessels have been identified [14] , [15] . In the tunica media, mesenchymal stem cells (MSC)-like cells can be isolated from SMC population, which express CD29 and CD44, and have multilineage potential for osteogenic and chondrogenic differentiation but not for adipogenic differentiation [16] , [17] . In adventitia, Sca-1 + progenitors can differentiate into SMCs and contribute to atherosclerosis of vein grafts in ApoE-deficient mice [18] . In addition, CD146 + perivascular MSC-like cells demonstrate osteogenic, chondrogenic and adipogenic potentials [19] . Furthermore, evidence exists that vascular endothelial cells (EC) can be converted into MSC-like cells by an activin-like kinase-2 receptor-dependent mechanism [20] . However, the characterization of these vascular progenitors is limited to nonspecific surface markers, and whether these vascular progenitors have an important role in the generation of proliferative or synthetic SMCs and the development of vascular diseases remains unclear. In this study, we isolate cells from the tunica media of the blood vessel wall and identify multipotent vascular stem cells (MVSCs) expressing markers such as Sox17, Sox10, S100β and neural filament-medium polypeptide (NFM). MVSCs can differentiate into MSC-like cells and subsequently SMCs. In addition, MVSCs and MSC-like cells respond differently to vascular growth factors. Importantly, lineage-tracing experiments show that MVSCs and proliferative or synthetic SMCs are not derived from mature SMCs. In response to vascular injury, MVSCs become proliferative and contribute significantly to vascular remodelling and neointima formation. These findings define a novel MVSC-MSC-SMC differentiation pathway, and support a new hypothesis that the differentiation of MVSCs instead of the de-differentiation of SMCs contributes to vascular remodelling and diseases. Identification and characterization of rat MVSCs First, we verified the existence of SM-MHC − cells in the tunica media by immunostaining the cross-sections of carotid arteries from Sprague Dawley (SD) rats for smooth muscle α-actin (SMA) and SM-MHC. As shown in Supplementary Fig. S1 , the majority of cells inside the elastic lamina layers were mature and contractile SMCs (SMA + /SM-MHC + ), whereas a small population (less than 10%) were negative for SM-MHC in the tunica media. We then isolated and characterized the cells from the tunica media of carotid arteries of SD rats. Using enzymatic digestion, we obtained a mixed cell population including both mature SMCs and non-SMCs. The mature SMCs had SM-MHC and calponin-1 (CNN1) assembled into stress fibres and were non-proliferative (negative for Ki67) ( Fig. 1a–c ). By contrast, the SM-MHC − cells were smaller, had no SM-MHC, CNN1 or SMA in stress fibres, expressed low level of SMA, and were highly proliferative ( Fig. 1b–c ). After being cultured in DMEM with 10% fetal bovine serum (FBS) for 3 days, the SM-MHC − cells started to multiply ( Supplementary Fig. S2 ) and eventually dominated the culture. 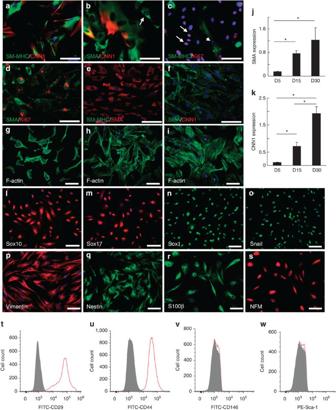Figure 1: Characterization of SM-MHC − cells isolated from rat carotid arterial tunica media. (a–c) Cells were isolated from arterial tunica media using enzymatic digestion method. The derived cells were immunostained for SMA, SM-MHC, CNN1 and Ki67 after being cultured in DMEM with 10% FBS for 3 days. Arrow in (b) indicates a SM-MHC−cell. Arrows in (c) indicate proliferating SM-MHC−cells in culture. Arrowhead in (c) indicates a non-proliferative mature SMC. (d–f) Cells were isolated from arterial tunica media using tissue explant culture method. The derived cells were immunostained for SMA, Ki67, SM-MHC and CNN1 after being cultured in DMEM with 10% FBS for 3 days. (g–k) SM-MHC−cells were cultured in DMEM with 10% FBS for 5, 15 and 30 days, and either subjected to fluorescein isothiocyanate-phalloidin staining for F-actin (g–i) (Nuclei were stained with DAPI) or used for qPCR to measure the gene expression of SMA and CNN1 (j–k). 18S ribosomal RNA was used to normalize the relative expression levels. Data were shown as average±standard deviation (n=3). * indicates significant difference between indicated groups using Holm'st-test. (P<0.01). (l–s) Immunostaining of isolated SM-MHC−cells cultured in DMEM with 10% FBS for 3 days for various markers, including Sox10, Sox17, Sox1, Snail, vimentin, nestin, S100β and NFM. (t–w) Flow cytometry analysis of SM-MHC−cells derived from arterial tunica media cultured in DMEM with 10% FBS for 3 days with antibodies against CD29, CD44, CD146 and Sca-1. Filled grey curves represent negative control samples; red curves represent samples stained with antibodies against CD29 (t), CD44 (u), CD146 (v) or Sca-1 (w). Scale bars, 100 μm. Figure 1: Characterization of SM-MHC − cells isolated from rat carotid arterial tunica media. ( a – c ) Cells were isolated from arterial tunica media using enzymatic digestion method. The derived cells were immunostained for SMA, SM-MHC, CNN1 and Ki67 after being cultured in DMEM with 10% FBS for 3 days. Arrow in ( b ) indicates a SM-MHC − cell. Arrows in ( c ) indicate proliferating SM-MHC − cells in culture. Arrowhead in ( c ) indicates a non-proliferative mature SMC. ( d – f ) Cells were isolated from arterial tunica media using tissue explant culture method. The derived cells were immunostained for SMA, Ki67, SM-MHC and CNN1 after being cultured in DMEM with 10% FBS for 3 days. ( g – k ) SM-MHC − cells were cultured in DMEM with 10% FBS for 5, 15 and 30 days, and either subjected to fluorescein isothiocyanate-phalloidin staining for F-actin ( g – i ) (Nuclei were stained with DAPI) or used for qPCR to measure the gene expression of SMA and CNN1 ( j – k ). 18S ribosomal RNA was used to normalize the relative expression levels. Data were shown as average±standard deviation ( n =3). * indicates significant difference between indicated groups using Holm's t -test. ( P <0.01). ( l – s ) Immunostaining of isolated SM-MHC − cells cultured in DMEM with 10% FBS for 3 days for various markers, including Sox10, Sox17, Sox1, Snail, vimentin, nestin, S100β and NFM. ( t – w ) Flow cytometry analysis of SM-MHC − cells derived from arterial tunica media cultured in DMEM with 10% FBS for 3 days with antibodies against CD29, CD44, CD146 and Sca-1. Filled grey curves represent negative control samples; red curves represent samples stained with antibodies against CD29 ( t ), CD44 ( u ), CD146 ( v ) or Sca-1 ( w ). Scale bars, 100 μm. Full size image With the tissue explant culture method, which relies on cell migration, only migratory and proliferative cells can be isolated. The cells migrating out of the tunica media expressed Ki67 and low levels of SMA, but did not express SM-MHC or CNN1 ( Fig. 1d-f ). These cells had the same characteristics as the SM-MHC − cells isolated using the enzymatic digestion method. In the previous literature, these SM-MHC − cells were defined as synthetic and/or proliferative SMCs [21] . However, a detailed characterization showed that the SM-MHC − cells exhibited significant changes in morphology, during the culture for an extended period. As shown in Supplementary Fig. S3 , the size of cell nucleus and the spreading area of the cells increased significantly (greater than threefold) within a 30-day time period, accompanied by the increase of stress fibres ( Fig. 1g-i ) and the increased expression of SMA and CNN1 ( Fig. 1j-k ). These results suggest that the proliferative/synthetic SMCs might be derived from the spontaneous differentiation of SM-MHC − cells in the medium with 10% FBS. To thoroughly characterize these SM-MHC − cells at the early stage (day 3) of primary tissue explant culture, we screened protein-marker expression with over 50 antibodies ( Supplementary Table S1 ), and found that isolated SM-MHC − cells uniformly expressed markers including neural crest cell markers Sox10, Sox1, Snail, vimentin and nestin, endoderm marker Sox17, neural cell makers NFM, peripherin, Brn3a, Phox2b and glia cell marker S100β ( Fig. 1l–s ; Supplementary Table S1 ), and general MSC makers including CD29 and CD44 ( Fig. 1t,u ). In addition, these SM-MHC − cells were negative for CD146 and Sca-1 ( Fig. 1v,w ), suggesting that these cells were distinct from previously identified perivascular MSC-like cells [19] or Sca-1 + progenitors [18] , [22] . These cells were also negative for markers for EC and EC conversion-derived MSC-like cells, for example, CD31/PECAM1 and VE-cadherin [23] , as well as the endothelial progenitor cell and haematopoietic stem cell markers CD34, CD133, c-Kit and Flk-1 ( Supplementary Table S1 ). To maintain the phenotype of these SM-MHC − cells, we performed screening for maintenance medium, and found a modified medium for neural crest stem cell (NCSC) culture that could maintain the cell morphology and the expression of aforementioned markers in the SM-MHC − cells. The maintenance medium contained DMEM with 2% chick embryo extract, 1% FBS, and 20 ng ml −1 of basic fibroblast growth factor (bFGF), and was used to expand the cells for further analysis. We further determined whether they were capable of differentiating into ectodermal and mesodermal lineages by treating cells with specific differentiation induction media [24] , [25] , [26] , [27] , [28] . Indeed, these SM-MHC − cells were capable of differentiating into Schwann cells (positive for glial fibrillary acidic protein, GFAP + ), peripheral neurons (positive for neuron-specific class III β-tubulin, that is, TUJ1 + ), SMCs (SM-MHC + ), chondrocytes (alcian blue staining), adipocytes (oil red staining) and osteoblasts (alizarin red staining) ( Fig. 2a-f ). 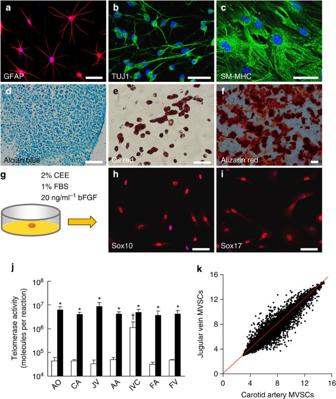Figure 2: Differentiation assay, single-cell cloning and telomerase activity assay of SM-MHC − cells derived from rat carotid arterial tunica media. (a–f) Staining of differentiated cell derived from SM-MHC−cells: Schwann cells for GFAP (a), neurons for TUJ1 (b), SMCs for SM-MHC (c), chondrocytes for aggrecan using alcian blue (d), adipocytes for lipid droplets using oil red (e) and osteoblasts for calcified matrix using alizarin red (f). Scale bars of (a–c) are 50 μm. Scale bars of (d–f) are 100 μm. (g) Schematic illustration of single-cell cloning with maintenance media. (h–i) Immunostaining of cloned MVSCs for Sox10 and Sox17. (j) Telomerase activity assay of MVSCs and the tissues from which MVSCs were isolated. The data was shown as average±s.d. (n=3). White bars indicate tissues, and black bars indicate isolated MVSCs. * indicates significant difference between MVSCs and the tissue from which the cells were derived using Student'st-test (P<0.05). † indicates significant difference between inferior vena cava and other blood vessels using Holm'st-test (P<0.05). AO, aorta, CA, carotid artery, JV, jugular vein, AA, abdominal artery, IVC, inferior vena cava, FA, femoral artery, FV, femoral vein. (k) DNA microarray analysis of MVSCs derived from rat carotid arteries and jugular veins (n=3). Figure 2: Differentiation assay, single-cell cloning and telomerase activity assay of SM-MHC − cells derived from rat carotid arterial tunica media. ( a – f ) Staining of differentiated cell derived from SM-MHC − cells: Schwann cells for GFAP ( a ), neurons for TUJ1 ( b ), SMCs for SM-MHC ( c ), chondrocytes for aggrecan using alcian blue ( d ), adipocytes for lipid droplets using oil red ( e ) and osteoblasts for calcified matrix using alizarin red ( f ). Scale bars of ( a – c ) are 50 μm. Scale bars of ( d – f ) are 100 μm. ( g ) Schematic illustration of single-cell cloning with maintenance media. ( h – i ) Immunostaining of cloned MVSCs for Sox10 and Sox17. ( j ) Telomerase activity assay of MVSCs and the tissues from which MVSCs were isolated. The data was shown as average±s.d. ( n =3). White bars indicate tissues, and black bars indicate isolated MVSCs. * indicates significant difference between MVSCs and the tissue from which the cells were derived using Student's t -test ( P <0.05). † indicates significant difference between inferior vena cava and other blood vessels using Holm's t -test ( P <0.05). AO, aorta, CA, carotid artery, JV, jugular vein, AA, abdominal artery, IVC, inferior vena cava, FA, femoral artery, FV, femoral vein. ( k ) DNA microarray analysis of MVSCs derived from rat carotid arteries and jugular veins ( n =3). Full size image The capability of the SM-MHC − cells differentiation into neural cells was also demonstrated in vivo . We isolated SM-MHC − cells from tunica media of carotid arteries of GFP rats, and transplanted them into a nerve conduit to bridge transected sciatic nerve, as described [25] . After 1 month, immunostaining of the longitudinal-sections showed that GFP labelled cells differentiated into Schwann cells and contributed to axon myelination, as evident by myelin basic protein expression ( Supplementary Fig. S4 ). These results indicate that these SM-MHC − cells in blood vessel wall are multipotent. Therefore, we defined these cells as MVSCs. MVSCs could be isolated from the tunica media of different blood vessels including jugular vein, aorta, abdominal artery, inferior vena cava, femoral artery and femoral vein beside carotid artery ( Supplementary Fig. S5 ), but not from adventitia layer, endothelium, or fat tissue around blood vessels using tissue explant culture method. Single-cell cloning and telomerase activity assay To further confirm the stemness of MVSCs, we performed a cloning assay ( Fig. 2g ). Dilutional cell cloning assay showed that the average plating efficiency of MVSCs was about 13%, and the cloned MVSCs retained the marker expression, as described in Supplementary Table S1 , including Sox10, Sox17 ( Fig. 2h-i ) and other MVSC markers (as exemplified in Supplementary Fig. S6a–f ), and could self-renew and maintain the multipotency ( Supplementary Fig. S6g–l ). To determine whether MVSCs had the capability to form neural spheres as neural crest cells [24] , [25] , [29] , rat MVSCs derived from cloning assay were cultured on ultralow-attachment plates. Indeed, MVSCs formed neural sphere-like aggregates ( Supplementary Fig. S7a ), and the cells within the spheres retained the expression of the MVSC markers such as Sox17, vimentin, SMA, nestin and S100β ( Supplementary Fig. S7b-f ). We then determined whether blood vessels and isolated MVSCs possess telomerase activity. Surprisingly, all blood vessels examined had telomerase activity, suggesting the presence of stem cells in the vascular wall ( Fig. 2j ). The isolated MVSCs had a marked increase (>100 fold) of telomerase activity compared with the respective vascular tissues from which the cells were isolated, suggesting the enrichment and purification of stem cells from vascular tissues, during the cell isolation process. Furthermore, we found no significant difference in telomerase activity in MVSCs isolated from different blood vessels. We used carotid artery and jugular vein as representatives to further compare the MVSCs from different blood vessels. DNA microarray showed that MVSCs from carotid arteries and jugular veins were almost identical ( Fig. 2k ), whereas only 3.6% of genes in expression showed significant difference of more than twofold ( Supplementary Table S2 ), suggesting that MVSCs derived from arteries and veins were similar. DNA microarray also showed that MVSCs expressed non-specific MSC markers such as CD29, CD44, CD73 and CD90 ( Supplementary Table S3 ). MVSCs did not arise from the de-differentiation of SMCs Our results suggest that previously identified proliferative/synthetic SMCs could be MVSCs and/or their derivatives following spontaneous differentiation in regular culture media. To directly determine whether MVSCs were derived from the de-differentiation of mature SMCs, we performed lineage tracing using SM-MHC as a marker in the SM-MHC-Cre/LoxP-enhanced green fluorescence protein (EGFP) mice [30] , [31] , [32] . Immunostaining showed that less than 10% of the cells in the carotid arterial tunica media of SM-MHC-Cre/LoxP-EGFP mice were not labelled with EGFP, indicating the existence of a small population of non-SMCs in the tunica media ( Fig. 3a ), consistent with the observation in the rat model ( Supplementary Fig. S1 ). Immunostaining for Cre and EGFP further showed that the EGFP − cells did not express Cre ( Supplementary Fig. S8 ). 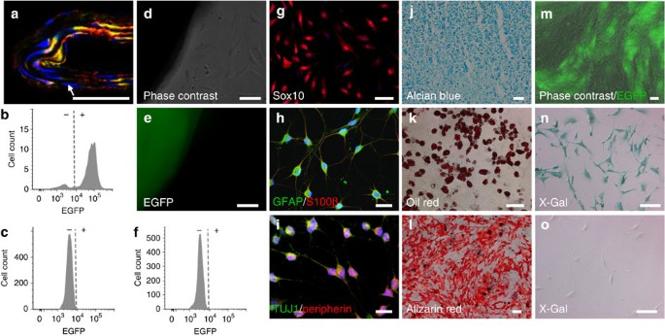Figure 3: Characterization of MVSCs derived from mouse blood vessels using lineage-tracing model with SM-MHC and Wnt1 as markers. (a) A cross-section of carotid artery from SM-MHC-Cre/LoxP-EGFP mouse was immunostained for EGFP (green) and SMA (red). The arrow indicates a SM-MHC−cell inside tunica media. Scale bar, 50 μm. (b,c) Flow cytometry analysis for EGFP of cells derived from carotid arteries of SM-MHC-Cre/LoxP-EGFP mice using enzymatic digestion method at day 0 (b) (n=3) and day 10 (c) (n=3), with the cells cultured in DMEM with 10% FBS. − indicates EGFP− population; + indicates EGFP+ population. (d,e) Phase contrast and fluorescent images of tissue explant culture of carotid arterial tissue from SM-MHC-Cre/LoxP-EGFP mice. Scale bars, 100 μm. (f) Flow cytometry analysis for EGFP expression in the cells derived in (d,e) (n=6). − indicates EGFP− population; + indicates EGFP+ population. (g) Immunostaining of the EGFP−cells derived from carotid arteries of SM-MHC-Cre/LoxP-EGFP mice for Sox10. Scale bar, 100 μm. (h–l) Staining of differentiated cells derived from EGFP−cells: Schwann cells for GFAP and S100β (h), neurons for TUJ1 and peripherin (i), chondrocytes for aggrecan using alcian blue (j), adipocytes for lipid droplets using oil red (k) and osteoblasts for calcified matrix using alizarin red (l). Scale bars of (i,j), 50 μm. Scale bars of (k–m), 100 μm. (m) EGFP expression in MVSCs after being co-cultured with OP9-Delta1 cell line for 2 weeks. Scale bar, 50 μm. (n,o) X-Gal staining of MVSCs derived from carotid arteries (n) and jugular veins (o) of Wnt1-Cre/LoxP-lacZ mouse. Scale bars, 50 μm. Figure 3: Characterization of MVSCs derived from mouse blood vessels using lineage-tracing model with SM-MHC and Wnt1 as markers. ( a ) A cross-section of carotid artery from SM-MHC-Cre/LoxP-EGFP mouse was immunostained for EGFP (green) and SMA (red). The arrow indicates a SM-MHC − cell inside tunica media. Scale bar, 50 μm. ( b , c ) Flow cytometry analysis for EGFP of cells derived from carotid arteries of SM-MHC-Cre/LoxP-EGFP mice using enzymatic digestion method at day 0 ( b ) ( n =3) and day 10 ( c ) ( n =3), with the cells cultured in DMEM with 10% FBS. − indicates EGFP− population; + indicates EGFP+ population. ( d , e ) Phase contrast and fluorescent images of tissue explant culture of carotid arterial tissue from SM-MHC-Cre/LoxP-EGFP mice. Scale bars, 100 μm. ( f ) Flow cytometry analysis for EGFP expression in the cells derived in ( d , e ) ( n =6). − indicates EGFP− population; + indicates EGFP+ population. ( g ) Immunostaining of the EGFP − cells derived from carotid arteries of SM-MHC-Cre/LoxP-EGFP mice for Sox10. Scale bar, 100 μm. ( h–l ) Staining of differentiated cells derived from EGFP − cells: Schwann cells for GFAP and S100β ( h ), neurons for TUJ1 and peripherin ( i ), chondrocytes for aggrecan using alcian blue ( j ), adipocytes for lipid droplets using oil red ( k ) and osteoblasts for calcified matrix using alizarin red ( l ). Scale bars of ( i , j ), 50 μm. Scale bars of ( k–m ), 100 μm. ( m ) EGFP expression in MVSCs after being co-cultured with OP9-Delta1 cell line for 2 weeks. Scale bar, 50 μm. ( n , o ) X-Gal staining of MVSCs derived from carotid arteries ( n ) and jugular veins ( o ) of Wnt1-Cre/LoxP-lacZ mouse. Scale bars, 50 μm. Full size image With enzymatic digestion culture, majority (about 92%) of the cells isolated from the carotid arteries of SM-MHC-Cre/LoxP-EGFP mice were EGFP + cells ( Fig. 3b ). However, after being cultured and passaged in DMEM with 10% FBS for 10 days, all the cells in culture were EGFP − ( Fig. 3c ), indicating that these cells were not derived from mature SMCs. In addition, in tissue explant culture, migratory and proliferative cells were EGFP − in contrast to strong EGFP fluorescence in the arterial tunica media ( Fig. 3d,e ). Flow cytometry also confirmed that none of the derived vascular cells expressed EGFP, which indicated that proliferative and migratory cells isolated from tunica media of blood vessels were not derived from the de-differentiation of mature SMCs ( Fig. 3f ). The lack of EGFP expression in MVSCs was unlikely due to the suppression of Rosa26 promoter activity in cell culture [33] . When SM-MHC-Cre/LoxP-EGFP mice were generated using β-actin (instead of ROSA26) promoter to drive the EGFP expression, tissue explant culture showed that cells derived from these mice did not express EGFP, while vascular cells in the tissue explant expressed EGFP ( Supplementary Fig. S9 ). To determine whether these EGFP − cells were similar to rat MVSCs, immunostaining and differentiation assay were performed. Immunostaining showed that these EGFP − cells uniformly expressed the same MVSC markers including Sox10 ( Fig. 3g ), Sox17, Sox1, Snail, vimentin, S100β and NFM ( Supplementary Fig. S10 ). In addition, these cells could be induced to differentiate into Schwann cells (GFAP + /S100β + ), peripheral neurons (TUJ1 + /peripherin + ), chondrocytes (alcian blue + ), adipocytes (oil red + ) and osteoblasts (alizarin red + ) ( Fig. 3h–l ), which further confirmed that EGFP − cells in tunica media were MVSCs. To determine whether MVSCs could differentiate into mature SMCs and turn on EGFP expression, we activated Notch signalling by co-culturing EGFP − MVSCs with OP9-Delta1 feeder cells [34] . After 2 weeks of co-culture, majority of the MVSCs showed strong green fluorescence ( Fig. 3m ). Immunostaining for SM-MHC confirmed that MVSCs indeed differentiated into SM-MHC + SMCs ( Supplementary Fig. S11a-c ). The fact that EGFP could be turned on after MVSCs differentiated into SMCs further confirmed that MVSCs are not derived from de-differentiation of contractile SMCs. Interestingly, a small portion of the EGFP + cells expressed proliferation marker Ki67 ( Supplementary Fig. S11d-f ), suggesting that newly differentiated SMCs had not exit cell cycle yet. To test whether MVSCs could differentiate into mature SMCs and turn on EGFP expression in vivo , we embedded MVSCs in collagen gel on the outer surface of a nanofibrous vascular graft, and implanted the grafts into athymic rats by performing carotid artery anastomosis [35] , [36] . After 1 month, immunostaining of the cross-sections showed that a small portion of the cells expressed EGFP, suggesting that MVSCs could differentiate into mature SMCs in vivo ( Supplementary Fig. S12 ). Previous lineage-tracing experiments showed that neural crest cells only contributed to the development of carotid artery, aortic arch and large arteries close to the heart [37] . To determine whether MVSCs from different vascular beds were derived from neural crest, we isolated MVSCs from arteries and veins in Wnt1-Cre/LoxP-LacZ mice. MVSCs derived from carotid arteries showed positive X-Gal staining whereas cells derived from jugular veins were negative ( Fig. 3n–o ), indicating that MVSCs are not necessarily derived from the neural crest origin. MVSCs-MSC-SMC differentiation pathway As shown in Figs 1 , 2 , 3 , MVSCs could differentiate into SMCs, and the cells at various stages of differentiation could contribute to the heterogeneity of SMCs. It is also possible that previously identified MSC-like cells could be derived from MVSCs. Therefore, we examined the spontaneous differentiation of MVSCs by culturing the freshly isolated MVSCs for 8 weeks in DMEM with 10% FBS. As shown in Fig. 4a,b , MVSCs were negative for CNN1 and SM-MHC. After 3 weeks, MVSCs expressed CNN1 but lost the nuclear expression of Sox17 (Sox17 − /Sox10 + /CNN1 + /SM-MHC − ) ( Fig. 4c-d ). At this stage, the cells lost the capability of differentiating into peripheral neurons and Schwann cells, but retained the potential for SMC, ostogenic, chondrogenic and adipogenic differentiation, similar to previously reported MSC-like cells. These results suggested that MVSCs could be the precursor of MSC-like cells identified in blood vessel by previous studies [16] , [17] , [38] . 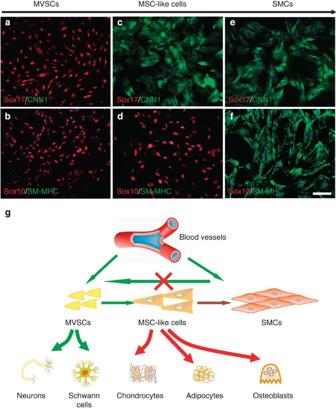Figure 4: Spontaneous differentiation of MVSCs into MSC-like cells and SMCs. (a–f) MVSCs were cultured in DMEM with 10% FBS for 5 days (a,b), 3 weeks (c,d) and 8 weeks (e,f), and were immunostained for Sox17, CNN1, SM-MHC and Sox10. Scale bar, 100 μm. The nuclei were stained with DAPI. (g) Schematic illustration of the spontaneous differentiation of MVSCs and the differentiation potential of the cells at different stages. Figure 4: Spontaneous differentiation of MVSCs into MSC-like cells and SMCs. ( a – f ) MVSCs were cultured in DMEM with 10% FBS for 5 days ( a , b ), 3 weeks ( c , d ) and 8 weeks ( e , f ), and were immunostained for Sox17, CNN1, SM-MHC and Sox10. Scale bar, 100 μm. The nuclei were stained with DAPI. ( g ) Schematic illustration of the spontaneous differentiation of MVSCs and the differentiation potential of the cells at different stages. Full size image In addition, after being cultured in DMEM with 10% FBS for 8 weeks, the cells lost the expression of Sox17 and Sox10 and spontaneously differentiated into mature SMCs (CNN1 + /SM-MHC + ) ( Fig. 4e–f ). These cells also lost the differentiation potential into neural and mesenchymal lineages (summarized in Fig. 4g ). These results suggested that long-term culture in the medium containing 10% FBS resulted in the spontaneous differentiation of MVSCs into MSC-like cells and subsequently SMCs, and that the cells at the various stages of differentiation might explain the heterogeneity of SMCs. Differential response of MVSCs and differentiated cells MVSCs at different stages of differentiation might respond differently to the same stimulation in the vascular microenvironment. To address this issue, we compared the effects of three vascular growth factors on undifferentiated MVSCs and MSC-like cells (3-week differentiation), as an example. The vascular growth factors used in this study included bFGF, platelet-derived growth factors-B (PDGF-B) and transforming growth factor-β1 (TGF-β1). PDGF-B and bFGF increased the proliferation of both MVSCs and MSC-like cells, while TGF-β1 suppressed the proliferation of MVSCs ( Fig. 5a ). It was also noted that PDGF had more dramatic effect on the proliferation of MSC-like cells compared with MVSCs. 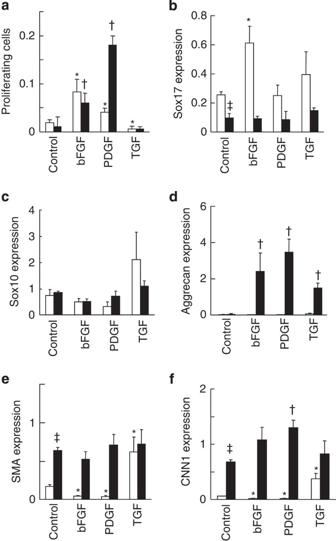Figure 5: Differential response of MVSCs and MSC-like cells to the treatment of vascular growth factors. The undifferentiated MVSCs (cultured in DMEM with 10% FBS for 5 days) and MSC-like cells (cultured in DMEM with 10% FBS for 3 weeks) were treated with 10 ng ml−1bFGF, 10 ng ml−1PDGF-B or 10 ng ml−1TGF-β1 for 24 h. White bars indicate undifferentiated MVSCs, and black bars indicate MSC-like cells. (a) EdU staining was used to quantify the proliferating cells. (b–f) qPCR analysis was used to quantify the gene expression of Sox17 (b), Sox10 (c), aggrecan (d), SMA (e) and CNN1 (f). 18S ribosomal RNA was used to normalize the relative expression levels. Data were shown as average±s.d. (n=3). * indicates significant difference between growth factors-treated and untreated MVSCs using Holm'st-test (P<0.05). † indicates significant difference between growth factor-treated and untreated MSC-like cells using Holm'st-test (P<0.05). ‡ indicates significant difference between MVSCs and MSC-like cells in absence of growth factors using Student'st-test (P<0.05). Figure 5: Differential response of MVSCs and MSC-like cells to the treatment of vascular growth factors. The undifferentiated MVSCs (cultured in DMEM with 10% FBS for 5 days) and MSC-like cells (cultured in DMEM with 10% FBS for 3 weeks) were treated with 10 ng ml −1 bFGF, 10 ng ml −1 PDGF-B or 10 ng ml −1 TGF-β1 for 24 h. White bars indicate undifferentiated MVSCs, and black bars indicate MSC-like cells. ( a ) EdU staining was used to quantify the proliferating cells. ( b – f ) qPCR analysis was used to quantify the gene expression of Sox17 ( b ), Sox10 ( c ), aggrecan ( d ), SMA ( e ) and CNN1 ( f ). 18S ribosomal RNA was used to normalize the relative expression levels. Data were shown as average±s.d. ( n =3). * indicates significant difference between growth factors-treated and untreated MVSCs using Holm's t -test ( P <0.05). † indicates significant difference between growth factor-treated and untreated MSC-like cells using Holm's t -test ( P <0.05). ‡ indicates significant difference between MVSCs and MSC-like cells in absence of growth factors using Student's t -test ( P <0.05). Full size image Quantitative PCR (qPCR) showed that MSC-like cells had much lower expression of MVSC marker such as Sox17 and higher expression of immature SMC markers such as SMA and CNN1 ( Fig. 5b,e,f ). bFGF significantly increased Sox17 expression while suppressed the expression of SMC markers including SMA and CNN1 of MVSCs ( Fig. 5b,e,f ), suggesting that bFGF might help maintain MVSCs at undifferentiated state. However, bFGF had no significant effect on the expression of Sox17, SMA and CNN1 but increased the synthesis of aggrecan ( Fig. 5d ) in MSC-like cells, suggesting that bFGF might promote a synthetic SMC phenotype in MSC-like cells. PDGF-B also suppressed the expression of SMC markers of MVSCs ( Fig. 5e,f ), but did not show any effect on Sox17 expression ( Fig. 5b ). In MSC-like cells, PDGF increased aggrecan synthesis and CNN1 expression, but had no effect on the expression of SMA ( Fig. 5d-f ). TGF-β1 significantly increased the expression of SMA and CNN1 in MVSCs ( Fig. 5e,f ), suggesting that TGF-β1 promoted MVSC differentiation into SMC lineage. In MSC-like cells, TGF-β1 promoted synthetic SMC phenotype by increasing the synthesis of aggrecan ( Fig. 5d ), similar to bFGF and PDGF. These results demonstrated the MVSCs and differentiated cells responded differently to vascular growth factors. MVSCs activation in vitro and in vivo Cell proliferation and expansion are important in the development of vascular diseases. Therefore, we performed in vitro and in vivo studies to determine the transition of MVSCs from quiescent state to proliferative state. We first isolated MVSCs from carotid arteries of SD rats using enzymatic digestion method. Within 24 h after cell isolation, immunostaining showed that MVSCs only expressed low levels of SMA, but not Sox10 or Ki67 ( Fig. 6a ), which indicated that MVSCs were quiescent in the blood vessels. However, after being cultured for another 24 h, MVSCs started expressing Sox10, as well as Ki67 ( Fig. 6b, c ), suggesting that MVSCs were activated and became proliferative. 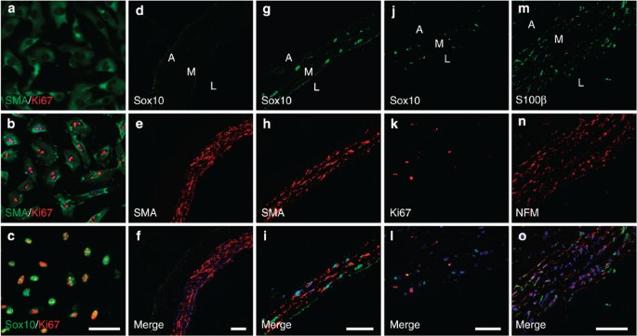Figure 6: MVSC activationin vitroandin vivo. (a–c) MVSCs were isolated from rat carotid arteries using enzymatic digestion method, and cultured in DMEM with 10% FBS for 24 h (a) and 48 h (b,c). The cells were immunostained for SMA, Ki67 and Sox10. Scale bar, 100 μm. (d–l) Immunostaining of cross-sections from native carotid arteries (d–f) and injured carotid arteries (day 5) (g–o) with the antibodies against Sox10, SMA, Ki67, S100β and NFM. A, Adventitia, L, Lumen, M, Media. The nuclei were stained with DAPI. Scale bars, 50 μm. Figure 6: MVSC activation in vitro and in vivo . ( a – c ) MVSCs were isolated from rat carotid arteries using enzymatic digestion method, and cultured in DMEM with 10% FBS for 24 h ( a ) and 48 h ( b , c ). The cells were immunostained for SMA, Ki67 and Sox10. Scale bar, 100 μm. ( d – l ) Immunostaining of cross-sections from native carotid arteries ( d – f ) and injured carotid arteries (day 5) ( g – o ) with the antibodies against Sox10, SMA, Ki67, S100β and NFM. A, Adventitia, L, Lumen, M, Media. The nuclei were stained with DAPI. Scale bars, 50 μm. Full size image Immunostaining also confirmed that the cells in the normal blood vessel wall did not express detectable level of MVSC markers (for example, Sox10, NFM or S100β) or proliferation marker Ki67 ( Fig. 6d–f , Supplementary Fig. S13a–f ), suggesting that MVSCs were quiescent under normal physiological conditions. In response to vascular endothelial denudation injury [39] , about 50% of cells inside the elastic lamina layers of arterial media were found expressing Sox10 at day 5 after injury ( Fig. 6g-i ), and about 40% of Sox10 + cells were positive for proliferative marker Ki67 ( Fig. 6j-l ). The percentage of proliferating cells is similar to what has been reported in the previous publications [40] , [41] , [42] . The Ki67 + cells were found only in Sox10 + MVSC population in tunica media, further confirming that MVSCs instead of SMCs could be activated to enter cell cycle on vascular injury. Of note, we also found Ki67-expressing cells in endothelial layer and adventitia layer after injury, indicating that ECs and adventitial cells were also activated to enter cell cycle for vascular remodelling. In addition, at day 5 after injury, the majority of the cells inside tunica media expressed MVSC cytoskeletal markers S100β and NFM ( Fig. 6m–o ), suggesting that MVSCs might have repopulated the tunica media following vascular injury and, possibly, SMC death. The difference in the relative percentage of Sox10 + cells and S100β + /NFM + cells in the tunica media could be explained by the difference in the temporal expression of these genes. MVSCs instead of SMCs contribute to vascular remodelling To further investigate the fate of SMCs after vascular injury, we performed endothelial denudation injury in the carotid artery of SM-MHC-Cre/LoxP-EGFP mice. Immunostaining showed that the cells in native carotid artery express EGFP but not MVSC marker S100β ( Fig. 7a-c ). Surprisingly, at day 5 after injury, the majority of the cells in tunica media expressed S100β instead of EGFP ( Fig. 7d-f ), which is consistent with previous notion that most SMCs may die by apoptosis while remaining cells proliferate and repopulate tunica media after vascular injury [43] , [44] . Although a low number of EGFP + cells were found at this time point, none of them expressed proliferation marker Ki67 ( Supplementary Fig. S14 ), which further confirmed that mature SMCs were not able to de-differentiate to entry cell cycle. Thus, MVSCs, rather than SMCs, were activated and proliferated rapidly to repopulate the tunica media after injury and contributed to vascular remodelling. 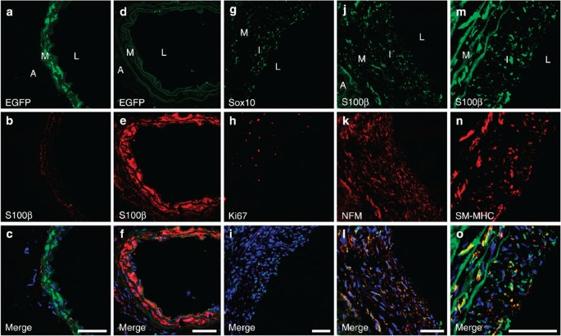Figure 7: MVSCs instead of SMCs contributed to vascular remodelling and neointima formation after endothelial denudation injury. (a–f) Immunostaining of cross-sections of native carotid arteries (a–c) and injured carotid arteries (day 5) (d–f) from SM-MHC-Cre/LoxP-EGFP mice with the antibodies against EGFP and S100β. (g–l) Immunostaining of cross-sections from carotid arteries of SD rats at day 15 after injury with the antibodies against Sox10, Ki67, S100β and NFM. (m–o) Immunostaining of cross-sections of carotid arteries from SD rats at day 30 after injury with the antibodies against S100β and SM-MHC. Scale bars, 50 μm. The nuclei were stained with DAPI. A, adventitia, I, intima, L, lumen, M, media. Figure 7: MVSCs instead of SMCs contributed to vascular remodelling and neointima formation after endothelial denudation injury. ( a – f ) Immunostaining of cross-sections of native carotid arteries ( a – c ) and injured carotid arteries (day 5) ( d – f ) from SM-MHC-Cre/LoxP-EGFP mice with the antibodies against EGFP and S100β. ( g – l ) Immunostaining of cross-sections from carotid arteries of SD rats at day 15 after injury with the antibodies against Sox10, Ki67, S100β and NFM. ( m – o ) Immunostaining of cross-sections of carotid arteries from SD rats at day 30 after injury with the antibodies against S100β and SM-MHC. Scale bars, 50 μm. The nuclei were stained with DAPI. A, adventitia, I, intima, L, lumen, M, media. Full size image The neointima formation was observed around day 15 after endothelial denudation injury in rat carotid arteries. Majority of the cells in the tunica media and neointima expressed MVSC makers including Sox10, NFM and S100β at day 15 and 30 ( Fig. 7g–l ; Supplementary Fig. S13g–l ), indicating that MVSCs were the major cell type in tunica media and neointima after vascular remodelling. In addition, the percentage of Ki67 + MVSCs inside the neointima was 32% at day 15, and decreased to less than 1% at day 30, suggesting a transient expansion of MVSCs in the vascular wall. Furthermore, around day 30, most of S100β + cells also expressed SM-MHC ( Fig. 7m-o ) and some of the cells were still proliferating, which is consistent with the in vitro observation ( Supplementary Fig. S11d–f ) that the newly differentiated SM-MHC + cells might have not exit cell cycle yet. At 1 month post-injury, alcian blue staining and Verhoeff's staining showed significant deposition of aggrecan and collagen I, respectively, in neointima populated by MVSCs ( Fig. 8a ; Supplementary Fig. S15a ), suggesting that MVSCs-derived cells had a synthetic phenotype and contributed to the matrix synthesis during neointima formation. Immunostaining showed that some of the MVSCs in neointima differentiated into chondrogenic cells (S100β + /collagen II + ) ( Supplementary Fig. S15b ), which demonstrated a novel mechanism of ectopic cartilage tissue formation in the injured blood vessels. 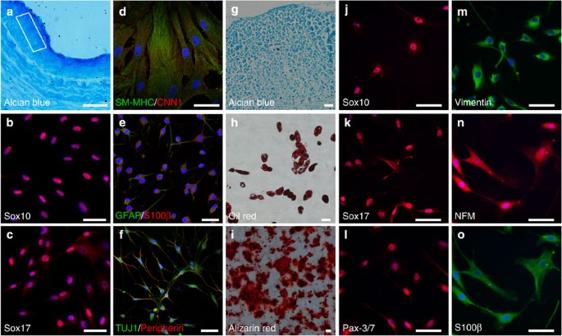Figure 8: Characterization of MVSCs from neointima in rat and MVSCs from normal human carotid artery. (a) Alcian blue staining of a cross-section of carotid artery from SD rat at week 5 after injury. Square indicates the area where the cells were isolated. Scale bar, 50 μm. (b,c) The cells isolated from neointima in rat were stained for MVSC markers Sox10 and Sox17. Scale bars, 50 μm. (d–i) The cells isolated from neointima were subjected to differentiation assays and stained for SMC markers SM-MHC and CNN1 (d), Schwann cell markers GFAP and S100β (e), neuronal marker TUJ1 and peripherin (f), aggrecan in chondrogenic culture using alcian blue (g), oil droplets in adipogenic culture using oil red (h), and calcified matrix in osteoblastic culture using alizarin red) (i). Scale bars of (d–f), 50 μm. Scale bars of (g–i), 100 μm. (j–o) Immunostaining of MVSCs isolated from human carotid arteries with antibodies against Sox10, Sox17, Pax-3/7, vimentin, NFM and S100β. Scale bars, 100 μm. Figure 8: Characterization of MVSCs from neointima in rat and MVSCs from normal human carotid artery. ( a ) Alcian blue staining of a cross-section of carotid artery from SD rat at week 5 after injury. Square indicates the area where the cells were isolated. Scale bar, 50 μm. ( b , c ) The cells isolated from neointima in rat were stained for MVSC markers Sox10 and Sox17. Scale bars, 50 μm. ( d – i ) The cells isolated from neointima were subjected to differentiation assays and stained for SMC markers SM-MHC and CNN1 ( d ), Schwann cell markers GFAP and S100β ( e ), neuronal marker TUJ1 and peripherin ( f ), aggrecan in chondrogenic culture using alcian blue ( g ), oil droplets in adipogenic culture using oil red ( h ), and calcified matrix in osteoblastic culture using alizarin red) ( i ). Scale bars of ( d – f ), 50 μm. Scale bars of ( g – i ), 100 μm. ( j – o ) Immunostaining of MVSCs isolated from human carotid arteries with antibodies against Sox10, Sox17, Pax-3/7, vimentin, NFM and S100β. Scale bars, 100 μm. Full size image To determine whether there were still undifferentiated MVSCs in neointima, we isolated cells from neointima tissue 1 month after injury, using the explant culture method. Indeed, cells with same marker expression and differentiation potential as MVSCs could be derived from neointima tissues ( Fig. 8b-i ), suggesting that MVSCs were capable of self-renewal in vivo during vascular remodelling. MVSCs exist in human blood vessels To test whether MVSCs exist in human blood vessels, we used human carotid artery as a representative, and characterized the cells isolated by tissue explant culture. Indeed, MVSCs could be isolated from human arteries, and the cells expressed MVSC markers such as Sox10, Sox17, Pax-3/7, vimentin, NFM and S100β ( Fig. 8j–o ). Similar to rodent MVSCs, human MVSCs can be induced to differentiate into Schwann cells, neuronal cells, SMCs, chondrocytes and adipocytes ( Supplementary Fig. S16 ). The identification of MVSCs brings a new perspective on vascular remodelling and disease development. Our in vitro experiments suggest that proliferative/synthetic SMCs are derived from the differentiation of MVSCs instead of the de-differentiation of mature SMCs. In vivo experiments also demonstrate that MVSCs, rather than mature SMCs, repopulate the tunica media and form neointima after endothelial denudation injury. These results provide the first direct evidence to support the MVSC differentiation hypothesis and disprove the SMC de-differentiation theory. The fact that highly expandable and migratory MVSCs were not derived from mature SMCs suggests that the previously reported decrease of contractile markers in SMC culture in vitro , or after vascular injury in vivo , could be attributed to the rapid expansion of MVSCs and their spontaneous differentiation into immature SMCs. MVSCs not only proliferate and differentiate, but also become synthetic and secrete matrix proteins such as collagen I, collagen II and aggrecan. The multipotential of MVSC differentiation into SMCs, chondrogenic cells and other lineages offers a novel and reasonable explanation for the complex phenotypes of cells in the diseased vessel. MVSCs at different stages of differentiation could also explain the heterogeneity of SMC in culture and in vivo . The fact that MVSCs and their derivatives respond differently to vascular growth factors underscores the importance of characterizing the cell culture from blood vessels. In the literature, the differentiation stage of SMCs is usually not well characterized. For example, the cells positive for SMA, SM-22α and CNN1 are often treated as SMCs, rather than immature SMCs or partially differentiated MVSCs. In many studies, the cells in culture may not be homogeneous at a specific differentiation stage, which may result in conflicting observations and explanation. Previous studies have identified a subpopulation of SMCs, termed 'epithelioid' cells, from newborn or injured vessels [45] , [46] , [47] , [48] . The origin of these SMCs is not known, and the relationship of 'epithelioid' cells with vascular stem cells has not been explored. It is very likely that 'epithelioid' SMCs are derived from MVSCs. However, in adults, MVSCs can be isolated from both normal vessels and injured vessels, but 'epithelioid' SMCs are only derived from injured vessels. It is possible that dormant MVSCs are a small population in normal vessels and may have been overlooked in previous studies. In addition to proliferative/synthetic SMCs, MVSCs could differentiate into mature SMCs (SM-MHC + ) in vitro and in vivo . It is also worth noting that the extent of MVSC activation, proliferation and differentiation could be dependent on the extent of vascular injury and SMC damage [42] . However, a recent study using SM-MHC as a marker for lineage tracing demonstrates that neointima contains proliferative cells derived from mature SMCs at 3 weeks following vascular injury [49] . There are two possible explanations for this apparent discrepancy. First, these proliferating cells could be derived from MVSCs after such a long time period. Indeed, we have shown that newly differentiated SMCs (SM-MHC + ) may not have exited the cell cycle completely ( Supplementary Fig. S11d–f ). In addition, at an earlier time point (for example, within a week), we never detected proliferating cells positive for SM-MHC ( Fig. 1c ). Second, the two transgenic mouse lines of SM-MHC-Cre, used for the lineage tracing of SMCs, were generated independently [30] , [50] . We cannot exclude the possibility that a subtle difference in the promoter of SM-MHC in these two mouse lines exists. Although both mouse lines have been verified with extensive characterization and should be appropriate for tracing the fate of mature SMCs, further studies are needed to directly compare these mouse lines. Another study on the lineage tracing of SMCs shows that SMCs give rise to osteogenic and chondrogenic cells in arteries [17] . However, SM22α instead of SM-MHC was used as the marker for lineage tracing in this study. Because SM22α is also expressed in MVSCs and their derivatives, this study may not distinguish the source of the cells between MVSCs and SMCs. Another important finding is that MVSCs are the cell type in tunica media that can be activated by vascular injury to proliferate and participate in remodelling. Neointima cells have a large cell body, secrete extracellular matrix (ECM) and express lower levels of the smooth muscle-specific contractile proteins [51] , which is consistent with our findings on the changes of cell morphology and the expression of SMC markers during the spontaneous differentiation of MVSCs. In this study, we showed that MVSCs, instead of SMCs, are the major cell type in neointimal tissue as characterized by MVSC makers. Given the fact that some MVSCs in neointima still retain multipotency, it is reasonable to propose that aberrant activation, expansion and differentiation of MVSCs may contribute to not only SMC differentiation and cartilage formation but also many other aspects of vascular diseases such as fat and cholesterol metabolism, matrix remodelling and calcification. As the rodent model of denudation injury does not result in significant fat and cholesterol accumulation and intima calcification, the possibility of MVSC differentiation into adipogenic and osteogenic cells in diseased vessels remains to be tested using atherosclerosis models. The identification of MVSC in human arteries makes MVSC a potential therapeutic target of vascular diseases. MVSCs in arteries and veins may have different developmental origins. Wnt1 lineage-tracing experiments suggest that MVSCs in carotid arteries may be neural crest origin. In contrast, for blood vessels not developed from neural crest (for example, jugular vein), MVSCs are negative for Wnt1. It is possible that these MVSCs are derived from other germ layers such as mesoderm. Nevertheless, MVSCs from carotid arteries and jugular veins have similar gene expression profile, suggesting that MVSCs in different vascular beds, regardless of their developmental origins, may share similar characteristics. In addition, MVSCs are different from NCSCs because MVSCs do not express some NCSC markers such as p75, HNK1, Slug or AP2 (refs 25 , 52 , 53 , 54 ). To date, MVSCs are a unique precursor identified for adult MSC-like cells, and MSC precursors similar to MVSCs probably exist in many other tissues. MVSCs express CD29 and CD44, two nonspecific surface markers of MSCs and SMCs. However, there was no specific marker, especially no transcriptional factor marker, for MSCs. In this study, we have identified several transcriptional markers and cytoskeletal markers in MVSCs, such as Sox17, Sox10, nestin, NFM and S100β. In addition, we showed that MSC-like cells were also positive for some of these markers (except Sox17). These results provide insight into the characteristics of MVSCs and MSC-like cells, not only in blood vessels, but also in other tissue types. This study supports a new hypothesis that MVSC activation and differentiation, instead of SMC de-differentiation, results in the proliferative and synthetic cells in the vascular wall, and that the aberrant activation and differentiation of MVSCs may play an important role in the development of vascular diseases. These findings provide unprecedented insight into the role of stem cells in vascular diseases and remodelling, which suggests that vascular diseases are stem cell diseases. These findings may have transformative impact on vascular biology and diseases, and may lead to new therapies using MVSCs as a therapeutic target. Generation of transgenic mice and genotyping Animal studies were approved by the ACUC committee at UC Berkeley, and were carried out according to the institutional guidelines. Transgenic mice, expressing Cre recombinase under the control of the SM-MHC promoter were mated with transgenic mice with a construct of Rosa26-LoxP-EGFP or Actin-LoxP-EGFP (Jackson laboratory) to generate SM-MHC-Cre/LoxP-EGFP mice. Transgenic mice, expressing Cre recombinase under the control of the Wnt1 promoter were mated with Rosa26-LoxP-LacZ mice to generate Wnt1-Cre/LoxP-LacZ mice. Genotyping was performed with PCR using total DNA extracted from mice tail tissues, as described previously [30] , [31] , [55] . The sequences of primers used for genotyping were shown in Supplementary Table S4 . Cell isolation Cells were isolated from the blood vessels in rat, mouse and human. Human carotid arteries were obtained from National Disease Research Interchange (Philadelphia, PA). The cell isolation methods were described previously [56] . Briefly, the tissue segments were washed three times with PBS supplemented with 1% penicillin/streptomycin (P/S). The surrounding connective tissues and adventitia were dissected away under a dissecting microscope. Endothelium was removed by scraping off the cell layer on the luminal surface with sterile scalpel blades. For tissue explant culture method, the tunica media was cut into mm size and placed onto the surface coated with 1% CellStart (Invitrogen) in 6-well plates. The cells were cultured in DMEM with 10% FBS (Thermo Fisher Scientific), or in DMEM with 2% chick embryo extract (MP Biomedical), 1% FBS, 1% N2 (Invitrogen), 2% B27 (Invitrogen), 100 nM retinoic acid (Sigma-Aldrich), 50 nM 2-mercaptoethanol (Sigma-Aldrich), 1% P/S and 20 ng ml −1 bFGF (R&D Systems) (maintenance medium). For enzymatic digestion methods, tissues were incubated with 3 mg ml −1 type II collagenase (Sigma-Aldrich) in DMEM with a 1/5 (w/v) ratio of tissue (g) to enzyme solution (ml). After incubation at 37 °C for 30 min, the same volume of 1 mg ml −1 elastase (Sigma-Aldrich) solution was added to the solution containing the tissue and collagenase. The tissues were incubated for another 1–2 h until all the tissues were digested. Cells were then seeded onto CellStart-coated dishes and maintained at 37 °C in an incubator with 5% CO 2 . Cell cloning assays For the clonal assays, MVSCs were detached, and the cells were resuspended with maintenance medium and filtered through membranes with 40-μm pore size to obtain single cells. Filtered cells were seeded onto CellStart-coated 96-well plates at the clonal density (1 cell per well) and cultured for 3 weeks at 37 °C in an incubator with 5% CO 2 . Sphere formation and differentiation assays For sphere formation assay, cell suspension was plated onto ultralow-attachment 6-well plates (Corning). at the density of 0.5×10 6 cells per well in the presence of maintenance medium for 1 week. The derived neural sphere-like aggregates were collected and embedded into optimal cutting temperature compound (Tissue Tek) for cryosectioning and immunostaining. For the directed differentiation of MVSCs into peripheral neurons, Schwann cells, osteoblasts, adipocytes and chondrocytes, the cells were incubated in specific induction media, described previously, for 1–3 weeks [24] , [25] . Telomerase activity assay Telomerase activities of MVSCs and the tissues from which the cells were isolated were measured using telomeric repeats amplification protocol combined with real-time detection of amplification products, using a Quantitative Telomerase Detection kit (US Biomax), according to the instruction of the manufacturer. Total protein extract (0.5 μg for each sample) was used in each reaction. Real-time PCR analysis was performed using an ABI PRISM 7,000 Sequence Detection System. The amount of molecules was quantified using the standard curve, and normalized with the level of α-actin in each sample measured by an ELISA kit (Cell Signaling Technology). Growth factor treatment and cell proliferation assay Undifferentiated MVSCs and partially differentiated MVSCs (cultured in DMEM with 10% FBS for 3 weeks) were starved in DMEM with 1% FBS for 24 h. followed by the treatment of 10 ng ml −1 bFGF (Peprotech), 10 ng ml −1 PDGF-B (Peprotech) or 10 ng ml −1 TGF-β1 (Peprotech) for another 24 h. The cell proliferation was quantified using Click-iT EdU Alexa Fluor 488 HCS Assay kit (Invitogen), according to the instruction of the manufacturer. RNA isolation for oligonucleotide microarray and qPCR MVSCs derived from carotid arteries and jugular veins of SD rats were lysed with Trizol reagent (Invitrogen). and total RNA was extracted as previously described [36] . For microarray analysis, the RNA pellet was resuspended in nuclease-free H 2 O and was subsequently diluted to a concentration of 0.50 mg ml −1 . Then, 10 μl of each sample was used for the analysis using an Affymetrix oligonucleotide microarray U133AA of Av2 chip containing 31,099 probe sets. Samples were labelled and hybridized according to Affymetrix protocols. Signal intensities were obtained for all probe sets and were organized using GeneTraffic version 3.2 microarray analysis software (Iobion). For qPCR, RNA pellets were resuspended in diethyl pyrocarbonate-treated H 2 O. Complementary DNA was synthesized using two-step reverse transcription with the ThermoScript RT–PCR system (Invitrogen), followed by qPCR with SYBR green reagent and the ABI Prism 7,000 Sequence Detection System (Applied Biosystems). The sequences of the primers used in this study are shown in Supplementary Table S5 . Carotid artery endothelial denudation model The rat and mouse carotid arteries were subjected to endothelial denudation injury as described previously [39] . Briefly, adult SD rats or transgenic mice were anaesthetized with isoflurane. Endoluminal injury to the left common carotid artery was produced by custom-made wire probes that consisted of a 10-cm long stainless steel wire soldered with a copper-beaded tip. Rats or mice were sacrificed at 5, 15 and 30 days after injury, with at least 6 animals for each time point. The blood vessels samples were rinsed with PBS and embedded in optimal cutting temperature compound for histological analysis. In vivo transplantation Electrospinning technique was used to produce vascular grafts and nerve conduits as previously described [25] , [35] , [36] , [57] . For cell transplantation into nerve conduits, MVSCs were isolated using tissue explant culture method from the carotid arteries of GFP rats. The cell suspension was mixed with cold matrigel solution at a 2:1 ratio (volume to volume), and injected into the nerve conduits. The tissue-engineered constructs were kept in the incubator for 1 h to allow gelation. The nerve conduit was inserted between the two nerve stumps and sutured, creating a gap of 1 cm between the two stumps. For the transplantation of MVSCs into microfibrous vascular grafts, MVSCs were derived from the carotid arteries of MHC-Cre/LoxP-EGFP mice using the tissue explant culture method. MVSCs were mixed with neutralized collagen solution (2 mg ml −1 ; diluted in MVSC maintenance medium), resulting in a cell density at 1 million cells per 0.5 ml. The collagen gel solution (with cells) was then used to fill in the space outside of the vascular graft in a 1-ml syringe and allowed to polymerize at 37 °C for 1 h. Then DMEM with 10% FBS containing 10 ng ml −1 TGF-β1 was added into the syringe to cover the grafts. After 1-day culture, the gel was contracted by the embedded cells and attached tightly onto the outer surface of the graft. The vascular grafts with cells were then transplanted into athymic rats using carotid artery anastomosis. Staining and histological analysis For immunostaining, cells or the tissue sections of blood vessels were fixed with 4% PFA, permeabilized with 0.5% Triton-100 (Sigma-Aldrich), and blocked with 1% BSA (Sigma-Aldrich). For actin cytoskeleton staining, samples were incubated with fluorescein isothiocyanate-conjugated phalloidin (Invitrogen) for 30 min to stain filamentous actin (F-actin). For the staining of other cell markers, samples were incubated with specific primary antibodies ( Supplementary Table S1 ) for 2 h at room temperature, washed with PBS for 3 times, and incubated with appropriate Alexa 488- and/or Alexa 546-labelled secondary antibodies (Molecular Probes). Nuclei were stained with 4,6-diamidino-2-phenylindole (DAPI) (Invitrogen). Fluorescence images were collected by a Zeiss LSM710 confocal microscope. For organic dye staining, cells or the tissue sections were fixed with 4% PFA for 30 min, washed and stained with alizarin red (Sigma-Aldrich), alcian blue (Sigma-Aldrich), oil red (Sigma-Aldrich) or Verhoeff's dye (American MasterTech) according to the instruction of the manufacturers. Images were collected by a Zeiss Axioskop 2 plus microscope. Flow cytometry analysis For flow cytometry analysis, cells were dissociated after the exposure to 0.2% EDTA for 20 min at room temperature. The cells in suspension were blocked with 1% BSA, incubated with specific primary antibodies, and then stained with secondary antibodies. Negative control sample was incubated with a nonspecific antibody with the same isotype as the specific primary antibody, and stained with the same secondary antibody. 7-AAD (BD Pharmingen) was used to exclude dead cells. Cells were analysed using FACScan flow cytometer (Becton Dickinson) and FlowJo software (Tree Star). Statistics Data were reported as means±s.d., unless otherwise indicated. All experiments were repeated at least three times. Comparisons among values for all groups were performed by one-way analysis of variance (ANOVA). Holm's t -test was used for the analysis of differences between different groups. Significance level was set as P <0.05. How to cite this article: Tang, Z. et al . Differentiation of multipotent vascular stem cells contributes to vascular diseases. Nat. Commun. 3:875 doi: 10.1038/ncomms1867 (2012).